Enhanced stochasticity of domain wall motion in magnetic racetracks due to dynamic pinning The problem of driven domain wall (DW) dynamics provides an excellent model system to study the general class of non-linear dynamical systems (for example, molecular transport at interfaces and surfaces, transport of energy in biological systems, microfluidics, etc). The role of defects and their influence on these dynamics is clearly of great importance. DW-based logic and memory devices [1] , [2] , which are lithographically fabricated into the shape of nanowires, are inevitably imperfect because of, for example, edge and surface roughnesses. Such defects, distributed within the nanowire, interact with the DW and give rise to a position dependence of the static DW energy. It follows that a finite driving force is needed to cause the DW to move and that this force clearly has a spatial dependence. The role of the imperfections, however, is much less clear when the DW is moving. The motion of a driven DW is mainly determined by its need to give up the energy gained from the driving force. It does so largely through damping. In this study, we present a detailed dependence of DW motion along nanowires on the strength of the driving magnetic field. We demonstrate that, as the DW motion changes from a translational to a precessional regime with increasing field, the DWs become more strongly pinned at localized pinning centers along the nanowire. We show that this is a result of the complex interaction between a driven DW and local imperfections, which greatly affects the DW dynamics, and can lead to enhanced stochasticity of the DW motion. Field-driven DW motion in spin-valve nanowires We explore the field-driven dynamics of DWs [3] , [4] , [5] , [6] , [7] , [8] , [9] , [10] in nanowires fabricated from spin-valves (SVs) comprised of CoFe/Cu/NiFeCo multilayers (see Methods ). The DW is created and travels within the SV's 'free layer'—the magnetically soft NiFeCo layer—so that the SV's resistance varies linearly with the position of the DW along the nanowire [11] , [12] , [13] ( Fig. 1 ). The variation in resistance is sufficiently large to enable single-shot, real-time measurements of the DW's trajectory [9] . The measurement procedure is as follows. First, a reset magnetic field (±150 Oe) is applied to orient the free layer's magnetization with the field (without changing that of the reference CoFe layer). Next, the field is set to a smaller value, below that needed to create any DWs in the free layer. This field serves as the driving force for DW propagation. A DW is then created in the free layer using a localized field generated from a nanosecond-long current pulse along an injection line (see Fig. 1 ) [7] . The injected DW very likely has a vortex structure [14] , [15] . The position and velocity of the DW between two electrical contacts spaced 22 μm apart along the SV is monitored from the temporal variation of the voltage measured between these contacts using a high-bandwidth oscilloscope and a small biased direct current. The latter is kept as small as possible while being sufficient to allow for single-shot voltage measurements. A value of ±2.0 mA was used, corresponding to a current density of ∼ ±2.5×10 7 A cm −2 in the free layer, after taking into account current shunting by the other layers in the spin valve. This current is too small to drive DW motion by itself in zero magnetic field through spin momentum transfer torque (SMT) [7] . However, its contribution to the DW's velocity in finite field is determined by measurements using currents of opposite polarities. 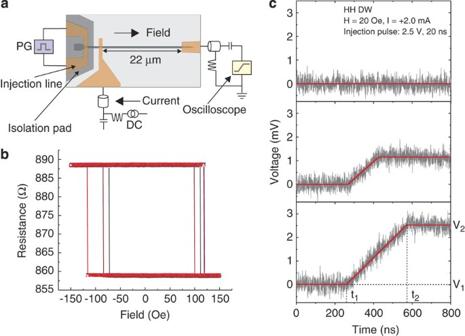Figure 1: Spin-valve nanowire domain wall (DW) detection scheme. (a) Schematic of the measurement setup. An 'injection' line, made of gold, is connected to a pulse generator (PG) for DW injection. Two electrical contacts, 22 μm apart, are placed on top of the nanowire. The left and right contacts are connected to a direct current source and a real-time oscilloscope through bias tees, respectively. The oscilloscope is used to measure the voltage signal induced by the DW motion in the free layer of the spin valve. (b) Resistance versus field loops of a spin-valve nanowire with a width of 200 nm. The switching field of the free layer varies for each measurement, owing to random fluctuations of the injection field that drives a DW from the large pad into the wire20. (c) Three representative voltage traces (thin grey lines) acquired by the oscilloscope, and fits to the traces (thick red lines). The injection pulse has an amplitude of 2.5 V and a duration of 20 ns. The driving field is 20 Oe and the bias current is +2.0 mA. The traces are recorded with a time resolution of 200 ps. The three traces represent the following situations in which the wall (i) stops before passing the left contact (upper panel), (ii) stops between the two contacts (middle panel) and (iii) travels all the way to the end of the wire.V1,V2,t1andt2are fitting parameters used to extract the DW velocity and displacement (with respect to the left contact). Figure 1: Spin-valve nanowire domain wall (DW) detection scheme. ( a ) Schematic of the measurement setup. An 'injection' line, made of gold, is connected to a pulse generator (PG) for DW injection. Two electrical contacts, 22 μm apart, are placed on top of the nanowire. The left and right contacts are connected to a direct current source and a real-time oscilloscope through bias tees, respectively. The oscilloscope is used to measure the voltage signal induced by the DW motion in the free layer of the spin valve. ( b ) Resistance versus field loops of a spin-valve nanowire with a width of 200 nm. The switching field of the free layer varies for each measurement, owing to random fluctuations of the injection field that drives a DW from the large pad into the wire [20] . ( c ) Three representative voltage traces (thin grey lines) acquired by the oscilloscope, and fits to the traces (thick red lines). The injection pulse has an amplitude of 2.5 V and a duration of 20 ns. The driving field is 20 Oe and the bias current is +2.0 mA. The traces are recorded with a time resolution of 200 ps. The three traces represent the following situations in which the wall (i) stops before passing the left contact (upper panel), (ii) stops between the two contacts (middle panel) and (iii) travels all the way to the end of the wire. V 1 , V 2 , t 1 and t 2 are fitting parameters used to extract the DW velocity and displacement (with respect to the left contact). Full size image Measurement of stochasticity of DW motion Histograms of the DW velocity and displacement in a succession of nominally identical measurements are depicted in Fig. 2a and b for various driving fields using a direct current of −2.0 mA. Results are shown for the propagation of head-to-head (HH) DWs, corresponding to the SV free layer switching from an antiparallel to a parallel alignment with the SV reference layer. In a small field of 2 Oe, the DW has a significant probability of getting trapped between the two electrical contacts, presumably because of local pinning sites in the nanowire. It appears from the histogram that there are two main pinning sites located at distances of ∼ 4 and 10 μm from the left contact. The DW velocity, on the other hand, exhibits a fairly narrow distribution. 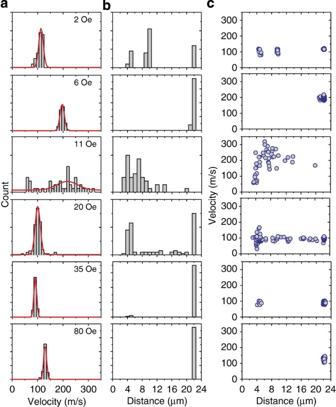Figure 2: Experimental measurement of stochastic nature of domain wall (DW) motion. Histograms of the velocity (a) and travelling distance (b) of the head-to-head (HH) wall in different fields. The biased direct current is −2.0 mA. The solid lines inaare Gaussian fits of the data. Panelcshows the plots of the DW velocity as a function of its travelling distance. As shown in Figure 2c , for this driving field of 2 Oe, the velocity is essentially independent of the DW displacement. For a larger field of 6 Oe, the DW almost always propagates to the end of the wire with a well-defined velocity. Interestingly, when the field is further increased to 11 Oe, the stochasticity of the DW motion is greatly enhanced: both the velocity and distance display much broader distributions. In most cases, the DW stops well before reaching the end of the wire. In addition, its velocity varies drastically from trace to trace. Subsequent increases in the field to 20, 35, and 80 Oe make the velocity and distance distributions narrower. For 80 Oe, the DW has 100% probability of reaching the end of the nanowire at a velocity of ∼ 130 m s −1 . Similar histograms were obtained for the opposite current polarity and for tail-to-tail (TT) DWs (not shown). Figure 2: Experimental measurement of stochastic nature of domain wall (DW) motion. Histograms of the velocity ( a ) and travelling distance ( b ) of the head-to-head (HH) wall in different fields. The biased direct current is −2.0 mA. The solid lines in a are Gaussian fits of the data. Panel c shows the plots of the DW velocity as a function of its travelling distance. Full size image The histogram of the DW velocity is fit by a Gaussian distribution, as shown by the solid lines in Fig. 2a . The most probable velocity obtained from the fit is plotted as a function of the driving field for the HH and TT walls in Fig. 3a and b , respectively. Results for both types of walls are very similar, although the data are offset by a small field of ∼ ±6 Oe, which most likely results from a small ferromagnetic coupling field between the free and reference layers. Taking into account this coupling field, the apparent DW propagation field is H p ∼ 9 Oe, slightly larger than that for similar nanowires made from a single permalloy layer [7] , and the Walker breakdown field (maximum of velocity) is H W ∼ 16 Oe. For both the HH and TT walls, the velocity is larger for negative current direction, consistent with a mechanism of current-assisted DW motion through SMT. However, the field dependence of the DW velocity is qualitatively the same for both current polarities at this current density. 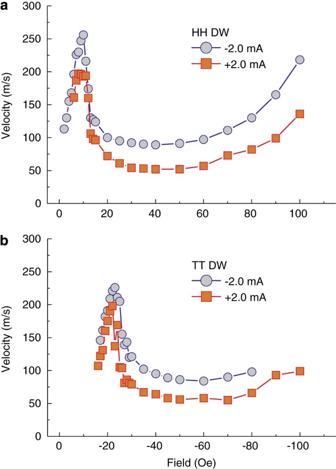Figure 3: Field dependence of domain wall (DW) velocity showing Walker breakdown field. Most probable DW velocity as a function of field for the head-to-head (HH) (a) and tail-to-tail (TT) (b) walls. The circles and squares correspond to biased direct currents of −2.0 mA and +2.0 mA, respectively. Figure 3: Field dependence of domain wall (DW) velocity showing Walker breakdown field. Most probable DW velocity as a function of field for the head-to-head (HH) ( a ) and tail-to-tail (TT) ( b ) walls. The circles and squares correspond to biased direct currents of −2.0 mA and +2.0 mA, respectively. Full size image The influence of imperfections in the nanowire on the DW velocity is reflected in the non-zero value of the propagation field H p ∼ 9 Oe. Below this value, the DWs cannot propagate over long distances, as they are pinned by local energy barriers. As shown in Figure 2 , for an applied field of 6 Oe (or ∼ 12 Oe, including the offset field), the DW propagates to the end of the wire with very high probability, which could imply that the driving field is large enough to overcome all local energy barriers along the wire. However, this cannot be the case, as for much larger applied fields (from 11 to 20 Oe), the DW is much more likely to be pinned, despite the larger driving field. Analytical model of DW motion To elucidate this paradoxical behaviour, we use a one-dimensional model of DW dynamics [15] , [16] . In this model, the DW dynamics are described by just two variables, the DW position, q , and the tilt angle of the DW's magnetization with respect to the nanowire's plane, which has the role of a conjugate momentum. Pinning along the nanowire is modelled by a periodic potential profile. In a real nanowire, the pinning potential originates, for example, from surface and edge roughness, and it is most likely neither uniform nor periodic. However, as shown below, the approximation of a periodic potential profile allows for a qualitative understanding of the DW dynamics in the presence of pinning. 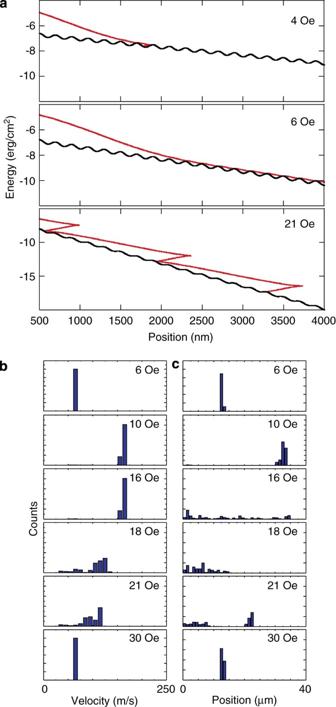Figure 4: Analytical model of domain wall (DW) motion in a periodic potential landscape. (a) DW energy versus position calculated for three different magnetic fields using the one-dimensional model of DW dynamics (red solid lines). The periodic pinning potential (taking into account the Zeeman energy) is shown as black solid lines. The DW is launched by an injection field of 200 Oe localized between 0 and 200 nm. (b–c) Histograms of the DW velocity (b) and propagation distance (c) obtained by varying the injection field between 195 and 205 Oe. Figure 4a shows the DW energy (red lines) and the potential profile (black lines) along the DW trajectory for applied fields of 4, 6 and 21 Oe. The Zeeman energy from the driving field adds a linear bias to the potential profile, with a slope proportional to the value of the field. As a result, the depth of the potential wells decreases for increasing fields until they are completely washed out, when the field reaches the static depinning field of 25 Oe. In the experiments, the DW is nucleated and launched into the nanowire by the local field generated by a voltage pulse. Not only does this field create the DW but it also provides the DW with an initial velocity. Although the detailed DW nucleation process at injection is complex and beyond the scope of our model, the 'launch' velocity is an important part of the problem and must be taken into account. In the model, the DW is launched with a large kinetic energy by a local injection field of 200 Oe (see Methods ). However, owing to the energy dissipation induced by Gilbert damping, the DW slows down as it moves away from the injection line. For H=4 Oe, the DW energy decreases to the point that the DW gets trapped in one of the pinning potential wells. For a slightly larger field (H=6 Oe), the rate at which the DW energy decreases is about the same as (or slightly slower than) that of the Zeeman energy change. Thus, the DW 'flies' over the pinning potential wells, even though this dynamic propagation field is much smaller than the static propagation field of 25 Oe needed to eliminate all the energy barriers. This is because the DW's momentum allows it to propagate despite non-zero energy barriers, because friction (that is, damping) is relatively small. Note that, as the damping is increased and the rate of dissipation of the DW's energy increases, the difference between the static and dynamic propagation fields decreases, until they are nearly identical in the quasi-static limit. When the field is further increased beyond the Walker breakdown field, the DW's instantaneous velocity increases and the gain in the Zeeman energy can no longer be dissipated by the Gilbert damping. As a result, a dynamical equilibrium cannot be reached, and the DW's magnetization starts to precess around the external field. As shown in Figure 4a , for an external field of 21 Oe, each rotation of the DW's magnetization by an angle, π , is associated with a backwards motion and a strong decrease of the kinetic energy of the wall. Depending on the phase of the pinning potential, the DW can then accelerate again or be trapped in one of the potential wells. In the example of Fig. 4a (bottom panel), the DW propagates during the first two π rotations of its magnetization, but is pinned at the end of the third one. Remarkably, the DW becomes more sensitive to pinning in this precessional regime, even though the driving field is much higher and the energy barriers preventing the wall's motion are much lower than in the low-field regime. Figure 4: Analytical model of domain wall (DW) motion in a periodic potential landscape. ( a ) DW energy versus position calculated for three different magnetic fields using the one-dimensional model of DW dynamics (red solid lines). The periodic pinning potential (taking into account the Zeeman energy) is shown as black solid lines. The DW is launched by an injection field of 200 Oe localized between 0 and 200 nm. ( b–c ) Histograms of the DW velocity ( b ) and propagation distance ( c ) obtained by varying the injection field between 195 and 205 Oe. Full size image Our model explains the origin of the enhanced stochasticity of the DW's propagation in the precessional regime. As shown in the bottom panel of Fig. 4a , the DW propagation becomes very sensitive to the relative phase between the pinning potential and the DW's precession. Thus, slight fluctuations in the wall's initial velocity can be magnified, leading to significant stochasticity in propagation distance and velocity. Histograms of the DW velocity and propagation distance are shown in Figure 4b and c for injection fields evenly distributed between 195 and 205 Oe. When the driving field is between the Walker breakdown field (15 Oe) and the static propagation field (25 Oe), both the wall's velocity and its propagation distance are widely distributed, in good agreement with experiments. We note that the concept of dynamic DW pinning has previously been inferred by studying the transmission probability of vortex DWs between two positions in a nanowire [10] or by measuring the different depinning fields of static and kinetic DWs at a notch [17] . Our experiments, in contrast, provide direct evidence that the DW is not necessarily pinned at the strongest pinning sites along the wire, as identified in small or zero fields, but rather the phase of the DW's oscillatory precession along the nanowire has a key role. As a result, the DW can become trapped at distinct sites along the entire length of the wire for a range of magnetic fields just above the Walker breakdown field. It is only because of the fact that we can directly detect in real time the position of individual DWs along the nanowire that we can reveal this phenomenon. In summary, our experiments and their interpretation using an analytical model show that it is the successive build up and release of energy from that stored within the DW's internal structure to that stored in the applied magnetic field that gives rise to the stochastic pinning of DWs for a special range of magnetic fields. Our finding has important implications for magnetic racetrack memory and logic devices. For instance, random pinning due to local imperfections in the racetracks is difficult to control and is deemed detrimental to maintaining the integrity of information coded in DWs as they propagate along the racetracks. Our results indicate that, however, a modest driving force of a moving DW in the translational mode may be sufficient to overcome very large energy barriers from imperfections. Thus, for example, the use of 'take-off' areas, strategically positioned along the racetracks, could allow DWs to 'fly over' regions that may, of necessity, contain unwanted pinning sites, such as from topology from structures related to reading or writing devices. Sample growth and device fabrication Spin-valve structures were deposited onto thermally oxidized silicon wafers by magnetron sputtering at ambient temperature. The layer sequence, from bottom to top, is as follows: 3 MgO/17.5 Ir 24 Mn 76 /3.5 Co 70 Fe 30 /2.4 Cu/1 Co 70 Fe 30 /20 Ni 65 Fe 20 Co 15 /1 Co 70 Fe 30 /1.5 Ru, where the numbers represent film thickness in nanometres. The bottom CoFe layer, which is pinned by exchange bias with the IrMn antiferromagnetic layer, forms the reference layer. The NiFeCo layer forms the free layer. The 1-nm thick CoFe interface layers are used to increase the giant magnetoresistance magnitude. After the film deposition, a combination of e-beam lithography, argon ion milling and optical lithography was used to pattern the films into nanowires, with widths varying from 50 to 600 nm. The nanowire has a large pad at the left end and a triangularly pointed tip at the right end (see Fig. 1a ). A DW injection line at the left side of the nanowire is electrically isolated from the nanowire by an alumina pad. Nanosecond-long voltage pulses along this line generate a local magnetic field that creates two DWs, one on each side of the injection line. The left DW is driven by the field towards the left and is outside of the detection region. The right DW, on the other hand, propagates towards the right and may enter the portion of the nanowire between the two electrical contacts. Measurement procedure For each histogram shown in Figure 2 , the experiment was repeated 150 times. In some cases, the DW stops moving before it passes the left contact (upper panel of Fig. 1c ). As a result, the DW velocity and distance cannot be determined. These data are not included in the histograms shown in Figure 2 . The voltage trace measured by the oscilloscope is fitted using: The amplitude of the trace V 2 – V 1 is proportional to the DW propagation distance. For large driving fields, the wall always reaches the end of the wire. Therefore, the traces taken in large fields may be used to calibrate the proportionality constant between the voltage amplitude and the DW displacement. The slope of the trace can then be used to calculate the DW velocity. Model details The DW position is at q =0 at time zero. The dynamical DW width is Δ =20 nm and the transverse anisotropy field is H k =1500 Oe. These two parameters are chosen to approximate a vortex DW [18] , which is the favored structure for the nanowire's dimensions [19] (thickness and width of 20 nm and 200 nm, respectively). Pinning along the nanowire is modelled as a periodic potential profile −( Vq 0 / π )cos(2 πq / q 0 ), where V =2.0×10 4 erg cm −2 and q 0 =200 nm are the depth and period of the pinning potential, respectively. Using these values, the static depinning field at which the energy barriers vanish is H dep = V / M S =25 Oe ( M S =800 emu cm −3 is the saturation magnetization of the wire). The Walker breakdown field used in the calculations is 15 Oe. Gilbert damping is α =0.02. The DW injection processes is modelled by an injection field H inj ∼ 200 Oe localized at 0< q < q inj =200 nm. This field, which is large enough to overcome the pinning potential, initiates the motion of the DW and provides it with its initial velocity. The DW propagation distance is calculated in a time span of 200 ns and this distance is used to determine its average 'time of flight' velocity. How to cite this article: Jiang X. et al . Enhanced stochasticity of domain wall motion in magnetic racetracks due to dynamic pinning. Nat. Commun. 1:25 doi: 10.1038/ncomms1024 (2010).